Atomic scale real-space mapping of holes in YBa2Cu3O6+δ The high-temperature superconductor YBa 2 Cu 3 O 6+ δ consists of two main structural units—a bilayer of CuO 2 planes that are central to superconductivity and a CuO 2+ δ chain layer. Although the functional role of the planes and chains has long been established, most probes integrate over both, which makes it difficult to distinguish the contribution of each. Here we use electron energy loss spectroscopy to directly resolve the plane and chain contributions to the electronic structure in YBa 2 Cu 3 O 6 and YBa 2 Cu 3 O 7 . We directly probe the charge transfer of holes from the chains to the planes as a function of oxygen content, and show that the change in orbital occupation of Cu is large in the chain layer but modest in CuO 2 planes, with holes in the planes doped primarily into the O 2 p states. These results provide direct insight into the local electronic structure and charge transfers in this important high-temperature superconductor. YBa 2 Cu 3 O 6+ δ (YBCO) has been extensively studied since its discovery, as it was the first material known to be superconducting above liquid nitrogen temperature. Although electron energy loss spectroscopy (EELS) [1] , [2] , [3] , [4] , [5] , [6] and X-ray absorption spectroscopy (XAS) [2] , [7] , [8] , [9] , [10] , [11] , [12] of YBCO compounds have been studied over the full range of oxygen stoichiometry, the presence of multiple, distinct copper and oxygen sites (see crystal structure in Fig. 1a ), each having different orbital symmetries and doping dependencies, give rise to complex spectra at the Cu L and O K edge. In these studies, the contributions to the spectra from different sites could not be spatially resolved, requiring reliance on the symmetry of the orbital occupation and their doping dependence to infer contributions to the spectra from different lattice sites. However, the conclusions drawn from these symmetry and doping arguments retain some ambiguity because the different Cu and O sites do not generally have unoccupied states with pure, well-defined symmetries (pure d x 2 −y 2 versus d y 2 −z 2 ) that can be neatly resolved as a function of photon polarization. Moreover, due to the strongly correlated nature of the cuprates, standard ab initio theoretical tools such as density functional theory capture some important details of electronic structure but have proven unreliable in predicting details of the cuprate electronic structure. Accordingly, a more complete description of the electronic structure of YBCO requires more direct means to distinguish the electronic structure of different sites. 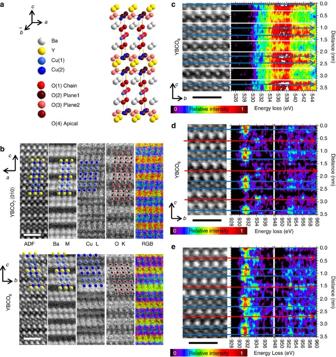Figure 1: Atomically resolved elemental maps and 2D representation of the OKand CuL2,3edges in YBCO. (a) The crystal structure of YBa2Cu3O7showing multiple, distinct atomic sites. (b) Atomic EELS elemental maps of YBCO7[010] (top) and YBCO6[100] (bottom) showing PCA-treated (10 components) maps of the BaM4,5, CuL2,3and OKedges. The coloured image is an RGB combination of Ba (blue), O (red) and Cu (green) maps. Spatially resolved EELS for (c) YBCO6at the OKedge, (d) YBCO6at the CuLedge and (e) YBCO7at the CuLedge. These spectra are integrated over the (ab) atomic planes but spatially resolved along thecaxis. The red, blue and white lines indicate the atomic planes corresponding to the chain layer (Cu(1)), CuO2plane layer (Cu(2), O(2,3)) and BaO planes (O(4)), respectively. Clear differences between the plane and chain layers are observed in the spectra. The scale bars are 1 nm. Figure 1: Atomically resolved elemental maps and 2D representation of the O K and Cu L 2,3 edges in YBCO. ( a ) The crystal structure of YBa 2 Cu 3 O 7 showing multiple, distinct atomic sites. ( b ) Atomic EELS elemental maps of YBCO 7 [010] (top) and YBCO 6 [100] (bottom) showing PCA-treated (10 components) maps of the Ba M 4,5 , Cu L 2,3 and O K edges. The coloured image is an RGB combination of Ba (blue), O (red) and Cu (green) maps. Spatially resolved EELS for ( c ) YBCO 6 at the O K edge, ( d ) YBCO 6 at the Cu L edge and ( e ) YBCO 7 at the Cu L edge. These spectra are integrated over the ( ab ) atomic planes but spatially resolved along the c axis. The red, blue and white lines indicate the atomic planes corresponding to the chain layer (Cu (1) ), CuO 2 plane layer (Cu (2) , O (2,3) ) and BaO planes (O (4) ), respectively. Clear differences between the plane and chain layers are observed in the spectra. The scale bars are 1 nm. Full size image In this report, we make use of recent developments in EELS resolution [13] , [14] , [15] , [16] to measure O K and Cu L 2,3 spectra in YBa 2 Cu 3 O 6+ δ with sufficient spatial and energy resolution to clearly distinguish the role of the planes and chains in real space. We show atomically resolved elemental maps for both doped and undoped YBCO as well as fine structure differences between chains and planes at both the Cu L and the O K edges. We demonstrate that, on doping YBCO from O 6 to O 7 , the atomically resolved data of the Cu L edge spectra in the planes remain very similar, whereas at the O K edge a lower energy peak arises corresponding to doped holes running through E F (consistent with the Zhang–Rice singlet band) and justifying the description of the cuprates as doped charge transfer insulators. Our results are contrasted with recent spatially resolved EELS measurements of YBCO:LSMO multilayers [17] , which exhibit a different O K edge energy dependence. In the chain layer, changes of spectral weight at the Cu L edge indicate that the additional dopant O transforms Cu from Cu 1+ to Cu 2+ . At the O K edge, a large transfer of spectral weight occurs as the doping is changed from O 6 to O 7 , from a high energy peak corresponding to empty chain states to a lower energy peak corresponding to full chain charge carrier states. The spatially resolved results are compared with polarized XAS data and shown to be largely consistent with the orbital symmetry assignments of the different Cu and O sites found in previous studies. Finally, we examine a novel means to explore the doping-dependent electronic structure of YBCO by modifying the O content through progressive electron beam exposure. Atomically resolved elemental maps Single crystals of YBa 2 Cu 3 O 6+ δ with two different oxygen stoichiometries ( δ= 0.03 and 0.97, hereafter referred to as YBCO 6 and YBCO 7 ) were measured. Figure 1b shows atomically resolved maps of YBCO 7 (top panel) taken in the ‹010› direction and YBCO 6 (bottom panel) with the corresponding scanning transmission electron microscopy (STEM) annular dark-field (ADF) image. These maps show that the chemical nature of the atomic sites in this complex structure can be readily identified and that the experimental mapping conditions are suitable to identify the edges of interest. Further maps are presented on Supplementary Fig. 1 . The oxygen atomic columns are clearly visible on the O K edge map. We note, however, that the oxygen (O(1)) atoms in the chains are not observed clearly in YBCO 7 , whether in the [100] or [010] directions. For the [010] projection, this might be linked to the presence of Cu in the same atomic column, whereas in the [100] projection, half the amount of oxygen present in the BaO and CuO 2 planes is present in the column, which might hinder the visibility. Furthermore, the contrast in oxygen atomic maps is strongly influenced by the neighbouring heavy atoms [18] . Doping dependent EELS in chains and planes Figure 1c presents the spatially resolved O K edge EELS spectra integrated over horizontal lines and plotted in a two-dimensional (2D) distribution in which the horizontal axis is the energy loss, the vertical axis is the position in the unit cell along the c axis, and the intensity is shown as a colour scale. The use of this representation to display EELS spectra provides a simple visualization of changes in the fine structure, layer by layer. The atomic resolution of our experiment in the c direction is confirmed, as differences can be seen between the plane and chain in this measurement geometry. This result will be discussed in detail further below by comparing the detailed spectra resolved in the different sites. On a similar 2D projection of the Cu L 2,3 edge of both YBCO 6 ( Fig. 1d ) and YBCO 7 ( Fig. 1e ), we can clearly resolve significant differences between the Cu L spectra in the chains and in the planes between doped and undoped YBCO, with further details visible in the detailed spectra shown in Fig. 2 . 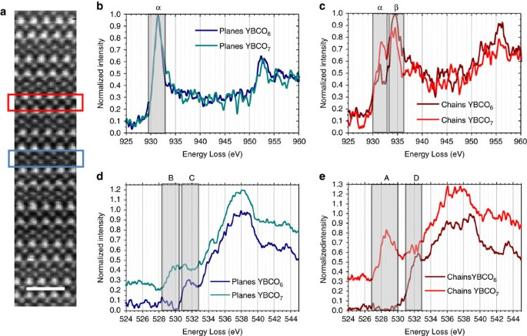Figure 2: Energy-loss near-edge structure of chains and planes in doped and undoped YBCO. (a) High-angle annular dark-field image showing the definition of the regions used for the chains and planes spectra (red rectangle and blue rectangle, respectively). Comparison of the raw CuL(b,c) and OK(d,e) between doped and undoped YBCO in planes (b,d) and chains (c,e) showing differences between the different electronic structures. Electronic transitions are marked as described in the text. Energy scales were aligned to data reported by XAS by Finket al.2Scale bar, 1 nm. Figure 2: Energy-loss near-edge structure of chains and planes in doped and undoped YBCO. ( a ) High-angle annular dark-field image showing the definition of the regions used for the chains and planes spectra (red rectangle and blue rectangle, respectively). Comparison of the raw Cu L ( b , c ) and O K ( d , e ) between doped and undoped YBCO in planes ( b , d ) and chains ( c , e ) showing differences between the different electronic structures. Electronic transitions are marked as described in the text. Energy scales were aligned to data reported by XAS by Fink et al. [2] Scale bar, 1 nm. Full size image Electronic structure differences at the Cu L edge To investigate the difference in the electronic structure between the planes and chains, the EELS spectra from the planes and chains are extracted from the spectrum images by summing pixels over the related area (see Fig. 2a ). To reduce the effect of beam exposure (discussed below), the spectra have been selected from the first two unit cells of the spectrum image in the case of YBCO 7 . In YBCO 6 , which is more stable, the signal could be averaged on identical atomic sites over 10 unit cells since no beam exposure dependence was seen. The Cu L 3 and L 2 white lines arise from transitions of 2p 3/2 → 3d 3/2 3d 5/2 and 2p 1/2 → 3d 3/2 , respectively. These edges are very sensitive to valence states as they are related to unoccupied states in the transition metal 3d band. The intensity of the Cu L edge from the chains is significantly lower than the one coming from the planes, as can be seen in Supplementary Fig. 2 . In YBCO 6 , the Cu L edge spectra in the plane layer ( Fig. 2b ) has a Lorentzian-like peak (labelled α) consistent with Cu 2+ (3 d 9 ), whereas the spectra in the chain layer is predominantly peaked at 934.5 eV (labelled β), similar to Cu 1+ in Cu 2 O (ref. 19 ). The small peak around 931.5 eV can be linked to residual oxygen in the chains forming Cu 2+ . These results are generally consistent with XAS and EELS studies of YBCO, as well as with other cuprates, such as La 2 −x Sr x CuO 4 (LSCO), that have only a CuO 2 plane layer [20] , [21] . (A comparison between polarization-dependent XAS and our spatially resolved EELS is provided in Supplementary Fig. 3 .) The polarization ( q )-dependent XAS (EELS) of spectra has been used to distinguish the planes and chains via the different orbital symmetries of the unoccupied states in the planes and chains. In contrast, the present measurements distinguish the planes and chains, and how they evolve with doping, much more directly, without any ambiguity due to the different Cu sites, and do so in real space. Of great significance, and once more without ambiguity due to the multiple sites, we demonstrate that, on doping YBCO from O 6 to O 7 , the atomically resolved data of the Cu L edge spectra in the planes remain very similar. However, the chain layer ( Fig. 2c ) exhibits a pronounced enhancement in intensity around 932 eV (slightly higher than the peak in the planes at 931.5 eV) and a reduction in intensity around 934.5 eV. This doping evolution is consistent with the additional electronegative O in the chain layer transforming the Cu in the chain layer from Cu 1+ to Cu 2+ (with the holes in the Cu 2+ of the chains occupying 3 d y 2 −z 2 symmetry states, as opposed to the 3 d x 2 −y 2 symmetry states of Cu 2+ in the planes). The doped oxygen is also well known to dope additional holes into the CuO 2 planes, with O 7 roughly corresponding to P =0.194 additional holes per CuO 2 plane [22] . However, according to previous XAS and EELS studies, these doped holes are understood to go primarily into the O 2 p states rather than the Cu 3 d orbitals, consistent with our measurements. Accordingly, the evolution of the Cu 3 d states in the planes is modest and is identified by a 3 d 9 L peak at ~932.5 eV that grows roughly linearly with doping [7] , [9] , [20] and is evident in the present experiments as a slight increase in intensity at 933 eV in the O 7 sample relative to the undoped O 6 sample ( Fig. 2b ). Electronic structure differences at the O K edge At the O K edge, the doping evolution of the O 2 p states in the planes is more pronounced than in the Cu L edge. In the plane layer ( Fig. 2d ), the EELS spectra of the O 6 sample has an onset of intensity at ~530 eV with a peak at ~531 eV (labelled C). When doped, a lower energy peak (labelled B) emerges corresponding to doped holes running through E F (consistent with the Zhang–Rice singlet band). This doping dependence is in accordance with the doping-dependent XAS and spatially integrated EELS of the pre-edge in LSCO [21] , [23] , the results demonstrate (1) that the doped holes locate predominantly into the O 2 p states (specifically with p x and p y symmetry [20] ) and (2) that the cuprates are strongly correlated systems (specifically doped charge transfer insulators), as evidenced by a transfer of spectral weight from the upper Hubbard band (UHB) (identified in our measurements as peak C) to states near the Fermi energy (peak B), rather than a simple band shift as one would have in a conventional insulator. In YBCO, a similar transfer of spectral weight of the two lowest energy pre-peaks is observed for XAS that, with light polarized along the a axis of the sample, is sensitive to the O 2 p x symmetry states [2] , [8] , [9] . The correspondence between our spatially resolved EELS of the plane layer and E // a XAS (see Supplementary Fig. 4 ) provides strong validation for the assignment of these E // a XAS pre-peaks to states in the planes and subsequently for the basic description of the cuprates as doped charge transfer insulators. This agreement is notable as our EELS of the plane layer differ markedly from the EELS of Chien et al. [17] on the YBCO planes in LSMO:YBCO multilayers, which show no discernable pre-peak structure and a broad peak at ~532.5 eV. The reason for these significant differences between the two studies is unclear, but they may be indicative of a difference in the basic electronic structure of YBCO in an LSMO:YBCO multilayer relative to a single crystal sample. In contrast, the O K spectra of the chain layer, discussed below, demonstrate a better qualitative agreement between our work and Chien et al. [17] , although the O doping of the sample in Chien et al. [17] is not known. In the chain layer ( Fig. 2e ), the O K edge EELS also exhibits a large transfer of spectral weight, with a peak at 532.5 eV (peak D) that diminishes and a lower energy peak at 529 eV (peak A) that emerges as the doping is changed from O 6 to O 7 . These spectral features can be identified with ‘empty’ (peak D) and ‘full’ (peak A) chain sites. Peak A has a clear correspondence with polarization-dependent XAS with the polarization along the b or c axes of the sample. 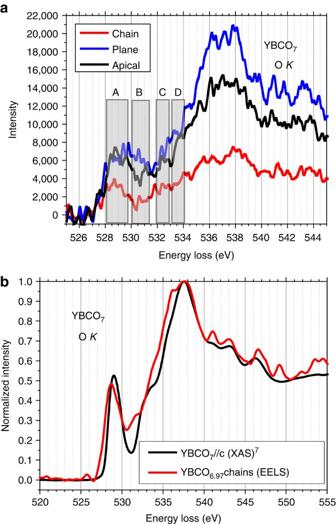Figure 3: EELS site-specific OKedge spectra and agreement with XAS. (a) Site-specific raw OKedge spectra of YBCO7per unit cell. (b) Comparison of XAS from ref.7and EELS using a convolution with a Gaussian distribution corresponding to the resolution of the EELS measurement. ( Figure 3b presents a scaled and Gaussian broadened comparison between XAS// c from ref. 7 and EELS of the chains in YBCO 7 , confirming this correspondence.) With these polarizations, XAS is sensitive to the O p y and p z symmetry orbitals, which are expected to be the lowest unoccupied orbitals of the O( 1 ) and O( 4 ) oxygen sites, respectively. Peak D, corresponding to empty chain states, however, is not very clearly identified on the basis of structural symmetry in polarization-dependent XAS. Here we show unambiguously that these states are identified with the chain layer and, more specifically, with the O(1) site. We can therefore infer from this new data that, on doping, supplementary holes in the planes, corresponding to the Zhang–Rice singlet, are going to states with oxygen character, whereas in the chains, hole charge carriers are formed with mixed contributions of Cu 2+ and p oxygen holes. This would suggest a charge transfer from the chain to the planes since no low-energy pre-peak is visible in the planes of YBCO 6 . Figure 3: EELS site-specific O K edge spectra and agreement with XAS. ( a ) Site-specific raw O K edge spectra of YBCO 7 per unit cell. ( b ) Comparison of XAS from ref. 7 and EELS using a convolution with a Gaussian distribution corresponding to the resolution of the EELS measurement. Full size image These spatially resolved measurements thus allow us to postulate more directly the localization of the charge and to identify the differences between the two compounds, due to the multiple inequivalent oxygen and copper sites, much more directly than the polarization-dependent XAS. Spatial resolution and comparison with polarized XAS The spatial resolution of the O K edge is examined in greater detail in Fig. 3a and in Supplementary Fig. 2 , in which the spectra are isolated into contributions from the O( 1 ) (chains), O( 2 , 3 ) (planes) and O( 4 ) (apical) sites. A similarity in the shape of the O K edge spectra corresponding to the chains and apical positions is clearly observed, indicating that the apical sites are associated with the chains rather than the planes. However, the finite spatial resolution of EELS spectrum image (SI) (with a Gaussian broadening due to the dynamics of the electron beam propagation of around 4 Å full width at half maximum) results in some contributions to the spectra at the apical O( 4 ) position from both chain O( 1 ) and plane O( 2 , 3 ) oxygen sites (see Supplementary Figs 5 and 6 ), limiting our ability to clearly distinguish such closely spaced atoms. As stated previously, the intensity of the Cu L edge from the chains is significantly lower than the one coming from the planes, as can be seen on Supplementary Fig. 2 . This might explain the differences compared with XAS measurements ( Supplementary Figs 3 and 4 ). Beam exposure induced doping dependence In addition to investigating the O 6 and O 7 end member samples, we also investigated the doping dependence of the EELS in YBCO by measuring the YBCO 7 sample as a function of exposure to the electron beam, which has for effect the removal of the loosely bound O( 1 ) intercalated interstitial oxygen from the chain layer (in contrast the O 6 sample, which has no O( 1 ) and is relatively insensitive to beam exposure). This experiment provides a novel means to investigate the doping dependence (converting YBCO 7 to YBCO 6+ δ ) of the electronic structure in the planes and chains by examining the EELS of YBCO 7 subject to different levels of beam exposure. On the O K edge ( Fig. 4a ), the beam exposure in the chains results in a reduction in peak A, associated with full chain states, and an enhancement in peak D, associated with ‘empty’ chains. In the planes, the beam exposure results in a transfer of spectral weight from the mobile carrier band (A) to the UHB states (B). Both of these observations are consistent with the beam exposure resulting in the removal of oxygen and subsequent reduction in the doping of the material. 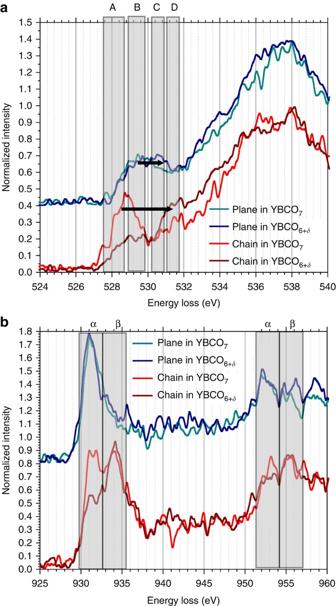Figure 4: Changes in the electronic structure of chains and planes during electron beam exposure. Effect of the loss of oxygen in the chains on the fine structures of the OK(a) and CuL(b) for planes and chains of YBCO7[100]. Spectra of planes have been shifted vertically for clarity. Arrows show charge transfer in planes (from the low-energy band to the UHB) and chains (from ‘full chain states’ to ‘empty chain states’) happening upon removal of chain oxygen through beam exposure. Figure 4: Changes in the electronic structure of chains and planes during electron beam exposure. Effect of the loss of oxygen in the chains on the fine structures of the O K ( a ) and Cu L ( b ) for planes and chains of YBCO 7 [100]. Spectra of planes have been shifted vertically for clarity. Arrows show charge transfer in planes (from the low-energy band to the UHB) and chains (from ‘full chain states’ to ‘empty chain states’) happening upon removal of chain oxygen through beam exposure. Full size image Similarly, on the Cu L edge ( Fig. 4b ), there is a modest change in the planes with beam exposure, which is not surprising given the relative insensitivity to doping previously seen. In the chain layer, however, peak α drops significantly and peak β increases slightly with beam exposure, consistent with the changes observed in Fig. 2c and roughly in agreement with a progressive reduction of the Cu( 1 ) from Cu 2+ to Cu + . Although the agreement between polarization-dependent XAS and our spatially resolved EELS is generally compelling, indicating a largely consistent understanding of the site-specific orbital occupation and symmetry in YBCO, there remain two notable discrepancies. First, from Fig. 2a (as well as Supplementary Fig. 6 ), the pre-peak corresponding to the hole states in the chains appears stronger at the side (close to the BaO( 4 ) layer) than in the centre of the chain (Cu( 1 )O( 1 ) atomic plane), suggesting that the holes are predominantly situated on the apical oxygen O( 4 ). This observation runs contrary to expectations for the formation of a 3 d z 2 −y 2 -symmetry Zhang–Rice singlet-like state forming around the Cu( 1 ) in the full chains. Accordingly, since the O( 1 ) is co-ordinated by two Cu( 1 ) atoms, whereas O( 4 ) is co-ordinated by only one Cu( 1 ) atom, it is expected that on a per-atom basis the hole occupation of O( 1 ) is larger than that of O( 4 ). This discrepancy may be associated with the shorter Cu( 1 )–O( 4 ) bond length (1.833 Å) relative to the Cu( 1 )–O( 1 ) bond (1.940 Å), and potentially a role of strong correlation effects altering the expected electronic structure. An additional consideration is related to the dynamics of electron scattering as the probe propagates in the sample, generating some contributions from adjacent sites, as shown recently in La 2 CuO 4 by Lugg and co-workers [24] . The second discrepancy relates to the presence of the peak β at 934.5 eV in the Cu L chain layer of fully doped YBCO 7 . This peak has been associated with empty chain sites, and polarization-dependent XAS measurements in YBCO 7 show no evidence for a peak at this photon energy [3] , yet the peak is present in the EELS spectra of the fully doped O 7 sample. This presence may indicate that beam exposure in the first two unit cells has already induced some O loss. However, that this peak evolves only very weakly with further beam exposure (underdoping) presents the possibility that it may yet be intrinsic. This possibility requires confirmation with further experiments at lower temperatures, and possibly at lower voltages, at which the mobility of species and knock-on effects can be reduced. In conclusion, by exploiting recent developments in electron microscopy, such as aberration correction, we are able to image the real-space electronic structure in the planes and chains of doped and undoped YBCO. These measurements directly show, in real space, the transfer of charge from the chain layer to the CuO 2 planes when the chains are intercalated with excess oxygen. Using EELS at the Cu L and O K edges, it is verified that the doped holes in the planes go primarily into the O 2 p rather than the Cu 3 d states, with an accompanying transfer of spectral weight from the UHB to a band of states near the Fermi energy as shown in La 2− x Sr x CuO 4 that have only a CuO 2 plane layer [20] , [21] , [23] . In contrast to the planes, the chain layer exhibits large changes at both the Cu L and O K edges, indicative of a change in valence from Cu 1+ to Cu 2+ in the chains. Together with symmetry-resolved but spatially integrated XAS measurements, a consistent description of the doping-dependent unoccupied states of YBCO is obtained. Sample preparation Single crystals of YBa 2 Cu 3 O 6+ δ with stoichiometries ( δ =0.03 and 0.97) were grown and detwinned, as described elsewhere [25] . Fresh TEM samples, in the [100] and [010] directions from the YBa 2 Cu 3 O 6.97 single crystal and one sample in the [100] using the YBa 2 Cu 3 O 6.03 crystal were prepared using an NVision 40 dual-beam focused ion beam (FIB) (Carl Zeiss AG, Germany) equipped with a 30-kV Ga + ion gun. The sample was thinned down to a relative thickness of t / λ =0.7 (where t is the absolute thickness and λ is the inelastic mean free path of the electrons in the TEM at the selected accelerating voltage of 80 kV and estimated at 20 nm) using progressively decreasing ion beam energies in the FIB down to 1 keV. This process was followed by Ar + milling with 900 eV ions at liquid nitrogen temperature using a Fischione Model 1040 NanoMill until a thickness of around 0.4 t/λ (that is, about 20 nm according to the mean free path estimator plugin for Digital Micrograph [26] ) was reached. The localized milling area obtained using this instrument helps reduce damage of the sample during thinning while cooling at LN 2 temperature. Experimental details EELS measurements were carried out on a FEI Titan 80–300 Cubed (Scanning) Transmission Electron Microscope ((S)TEM) (FEI Company, Eindhoven, The Netherlands) equipped with a high-brightness X-FEG electron source, aberration correctors for probe and image lenses, a monochromator and a high-resolution electron energy loss spectrometer 866 model Gatan Imaging Filter Tridiem. The experiments were performed at 80 keV in STEM mode where a fine probe of about 1 Å was rastered onto the specimen. The energy resolution was 0.7 eV, as the monochromator was not excited for this particular work. It is important to note that, to reduce ionization and oxygen removal from the chains, a very low electron beam current (<30 pA) was used. From each pixel, the high-angle scattered electrons were collected using a high-angle annular dark field detector while an EELS spectrum was recorded using the spectrometer. Dispersion and exposure time of 0.5 eV/channel and 0.05 s per pixel, respectively, were used for atomic mapping of the O K , Ba M and Cu L edges. The O K and Cu L edges’ fine structures were recorded in Spectrum Imaging mode using 0.1/channel and 0.2 eV/channel dispersions, respectively, and a collection time of 0.05 s per pixel. The spectrometer was tuned on the Ba M 4,5 edges. A collection angle of 82 mrad can be achieved in energy-filtered STEM mode, allowing most of the scattered electrons in the EELS entrance aperture. XAS data were taken from previously reported measurements by Hawthorn et al. [7] Data processing The 2D projection of the EELS spectrum from Fig. 1c–e and Supplementary Figs 5c and 6c were realized, summing the spectra from every pixel on each horizontal line to reduce the statistical noise and rebinning the spectrum image in the y direction ( c axis) by 2. Principal component analysis (PCA) was used for Fig. 1b and Supplementary Figs 1, 5b,d and 6b,d . A reconstruction using the first 10 principal components was performed using the weighted-PCA MSA Plugin [27] within Gatan Digital Micrograph software. The 2D projection of the EELS spectrum from Supplementary Figs 5d and 6d was realized summing the spectra from every pixel of the PCA-reconstructed data on each horizontal line to reduce the statistical noise. Spectra from Figs 2 and 3 , and Supplementary Figs 2c–f, 4a,b and 6a,b were obtained by decomposition of the Spectrum Image (SI) in atomic planes (each with the same number of pixels) and summing equivalent atomic sites over 3 unit cells. All spectra were aligned in energy using the Ba M 5 peak for SI containing Ba and this alignment was matched for high dispersion data of the O K edge. All spectra were normalized between 0 and 1. For comparison purposes a Gaussian broadening of 0.7 eV full width at half maximum was applied to the EELS and XAS spectra from Fig. 2d and Supplementary Figs 3 and 4 . How to cite this article: Gauquelin, N. et al. Atomic scale real-space mapping of holes in YBa 2 Cu 3 O 6 +δ . Nat. Commun. 5:4275 doi: 10.1038/ncomms5275 (2014).